Interface between path and orbital angular momentum entanglement for high-dimensional photonic quantum information Photonics has become a mature field of quantum information science, where integrated optical circuits offer a way to scale the complexity of the set-up as well as the dimensionality of the quantum state. On photonic chips, paths are the natural way to encode information. To distribute those high-dimensional quantum states over large distances, transverse spatial modes, like orbital angular momentum possessing Laguerre Gauss modes, are favourable as flying information carriers. Here we demonstrate a quantum interface between these two vibrant photonic fields. We create three-dimensional path entanglement between two photons in a nonlinear crystal and use a mode sorter as the quantum interface to transfer the entanglement to the orbital angular momentum degree of freedom. Thus our results show a flexible way to create high-dimensional spatial mode entanglement. Moreover, they pave the way to implement broad complex quantum networks where high-dimensionally entangled states could be distributed over distant photonic chips. The progress in technological developments over the last decades has enabled the realization of highly complex photonic quantum experiments [1] . A popular approach to increase the complexity of the set-up and the dimensionality of the observed system uses integration of optical elements on photonic chips. On these chips the most convenient way of encoding information is the path of the photons, which is inherently extendable to higher-dimensional systems [2] , [3] . Another possibility of encoding high-dimensional quantum information is the transverse spatial mode of light [4] . The fact that beams encoded with orbital angular momentum (OAM) can co-propagate along the same optical axes makes their use, especially over long distances, advantageous [5] , [6] , [7] , [8] , [9] . Various modes, such as OAM-carrying Laguerre-Gauss (LG) [10] , [11] , Ince-Gauss [12] and Bessel-Gauss [13] , have been used to demonstrate experimentally high-dimensionally entangled states and to implement quantum informational tasks. In a wide quantum network [14] , both degrees of freedom, local on-chip path encoding and long-distance bridging spatial modes, will have to be matched to each other. Recently, first experiments of an integrated OAM beam emitter demonstrated an interface between both fields, although not yet in the quantum regime [15] . In another approach, q-plates have been demonstrated to interface the OAM with the polarization of photons [16] , [17] . In this Article we demonstrate a quantum interface between two approaches to high-dimensional photonic quantum information: path encoding for complex on-chip experiments and OAM carrying light modes to transmit the information over large distances. At the same time, we investigate a flexible way to create higher-dimensional OAM entanglement that does not rely on angular momentum correlation. The essential tool in our experiment is a mode sorter (MS) that was invented [18] , [19] to convert the OAM content of an incident light beam to lateral positions of the output beam. By using this device in reverse, different spatial positions can be transformed to the cylindrically symmetric LG modes. We demonstrate that a high-dimensional path-entangled state can be transferred to high-dimensional OAM entanglement with the help of the reversed MS. Generation of OAM modes with a MS in reverse Transverse spatial LG modes have a helical phase front e ilθ , where l can take any integer value and represents the quanta of OAM each individual photon possesses [20] . If l ≠0, such modes exhibit a vortex along the beam axis and show a ring-shaped intensity structure; consequently they are also called ‘doughnut modes’. LG modes can be used to transmit more classical information [5] , [6] , [7] , [8] , [9] or realize a higher-dimensional quantum state [11] , [21] , [22] . To access the encoded information efficiently a MS was developed [18] , [19] , which consists of two freeform refractive optical elements that convert the OAM content of an incident light field to lateral positions of the output. The first element maps the azimuthal to the lateral coordinates. Thereby, the ring-shaped intensity is transferred to a straight intensity line and the l -dependent helical phase structure to a transverse phase gradient. The second element corrects for phase distortion due to optical path length differences. A lens after the second element Fourier-transforms the transverse phase gradient to specific spatial position, that is, finishes the sorting of the modes. Recently, the operation of the MS in reverse was demonstrated by converting a light field with a transverse phase gradient, which has been created with a spatial light modulator (SLM), into an LG mode [23] . Here we investigate a different, simple way of using the MS operated in reverse as a source for OAM states. A narrow slit that diffracts the light is positioned in the focal plane of the lens ( Fig. 1 inset). Thus, behind the lens, a parallel beam emerges with a phase profile given by the position of the slit relative to the optical axis. That phase distribution can be adjusted to be a multiple of 2 π by adjusting the lateral position of the slit. A subsequent MS in reverse transforms the state’s amplitude distribution into a circle and thus into an OAM state ( Fig. 1 inset). A continuous lateral movement of the slit leads to integer OAM modes at multiples of 2 π and fractional OAM in intermediate positions (see Fig. 1 and Supplementary Movie 1 ). To define the lateral position states, we overfill the slit with a Gaussian beam. Hence, the specific parameters of the slit define the characteristics of the OAM state generated. The width of the slit was chosen such that it corresponds approximately to the diffraction-limited spot size of a beam being focused by the lens just before the MS. The height of the slit defines the radial characteristics, but is not specifically controlled and larger than the beam radius in our experiment. As height is mapped to the radius (logarithmically) of the OAM beam generated, this will result in an OAM state with a corresponding radial extent. Additionally, hard apertures are present in the optical elements of the MS (see the inset in Fig. 1 ), which lead to diffraction of the transformed beam. Both, the unrestricted slit height and the apertures, result in an observation of higher-order radial modes containing the same OAM. A similar effect has been used in an experiment where OAM-containing Bessel beams have been separated by the MS in their azimuthal and radial components [24] . With our simple approach we were able to create LG modes up to order l =±10. The order of the generated modes was only limited by the size of the Gaussian laser beam used to illuminate the slit. Importantly, by using multiple slits superpositions of LG modes could also be generated [25] ( Fig. 2 ). 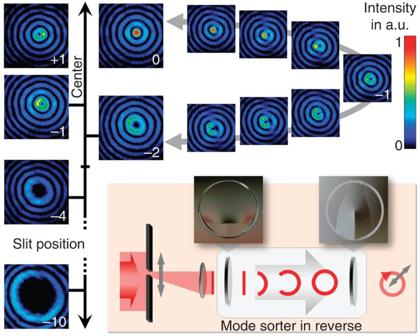Figure 1: Generation of OAM states from lateral position states. False colour images recorded with a CCD camera are shown for various OAM states up to the 10th order (white numbers). The distance between the lateral positions of the slit that generate integer OAM states was around 150 μm for the shown images. In between these positions, fractional OAM modes are generated. The multiple ring structure indicates the creation of higher-order radial modes containing the same OAM. It may be suppressed by shortening the length of the slit. Inset: Sketch of the set-up, where light is diffracted through a movable slit (width ~100 μm) positioned in the focal plane of a lens. It is transformed by two freeform refractive optical elements (MS—mode sorter in reverse) into different OAM states depending on the slit position (detailed description in the main text). Figure 1: Generation of OAM states from lateral position states. False colour images recorded with a CCD camera are shown for various OAM states up to the 10th order (white numbers). The distance between the lateral positions of the slit that generate integer OAM states was around 150 μm for the shown images. In between these positions, fractional OAM modes are generated. The multiple ring structure indicates the creation of higher-order radial modes containing the same OAM. It may be suppressed by shortening the length of the slit. Inset: Sketch of the set-up, where light is diffracted through a movable slit (width ~100 μm) positioned in the focal plane of a lens. It is transformed by two freeform refractive optical elements (MS—mode sorter in reverse) into different OAM states depending on the slit position (detailed description in the main text). 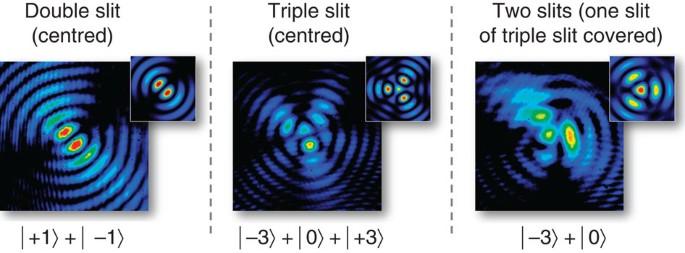Figure 2: Creation of superpositions of OAM states. If a double or triple slit is placed in front of the MS (Fig. 1inset) different superpositions of OAM modes are created (false colour images) depending on the slit dimensions and focusing parameters of the lens (see Methods). All imaged modes show reasonable qualitative agreement with the theoretical calculation of the expected superpositions (insets). Full size image Figure 2: Creation of superpositions of OAM states. If a double or triple slit is placed in front of the MS ( Fig. 1 inset) different superpositions of OAM modes are created (false colour images) depending on the slit dimensions and focusing parameters of the lens (see Methods). All imaged modes show reasonable qualitative agreement with the theoretical calculation of the expected superpositions (insets). Full size image To confirm that the generated annular-shaped modes have the correct helical phase, we modulate the generated modes with the opposite-handed phase holograms displayed on a SLM and investigate the resulting mode. First, we image the modulated mode with a charge-coupled device (CCD) camera. The recorded modal structure shows an intensity along the beam axis that resembles a fundamental Gauss mode or higher-order radial mode containing no OAM (see three exemplary tests in Fig. 3a ). In a second step, we unambiguously determine the OAM mode purity by adding a grating to the phase pattern on the SLM. We then couple the modulated first diffraction order into a single-mode fibre, thereby filtering higher-order components [10] , [26] . By additionally changing the phase holograms on the SLM, we are able to measure the efficiency with which the expected mode is generated and thereby the modal overlap between this mode and its neighbouring modes (see Fig. 3b ). Similar to the overlap if the interface is used for sorting [18] , we find an average overlap of 17±8% between the closest neighbouring modes, 5±4% between the second closest neighbours and 0.7±0.6% between the third closest neighbouring modes. Note that this performance might be improved by a recently introduced version of the MS scheme [27] . 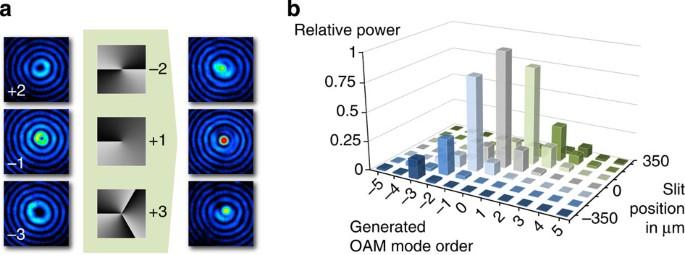Figure 3: Examination of the generated modes. (a) We use an SLM to modulate the generated mode (left side) with the opposite-handed phase hologram (phase modulation shown in grey scale, linearly from 0=black to 2π=white). The resulting intensities (right side) resemble the expected fundamental Gauss mode with an on-axis intensity maximum. However, a reduction of the modulated Gauss mode quality can be seen for higher orders. (b) We quantify these results by additional modulation of each generated mode (from −3rd order, dark blue, to 3rd order, dark green) with phase holograms of all neighbouring modes and coupling to a single-mode fibre (filtering higher-order modes). Thereby, we are able to measure the purity of the generated modes. We find that the expected OAM modes of a specific order are generated depending on the particular slit positions with high efficiency (highest bar for each slit position). The overlap with direct neighbouring modes is around 20%, which decreases down to <1% for third neighbours. The varying relative power for different orders stems from the Gaussian mode shape of the laser, through which the slit was moved. Figure 3: Examination of the generated modes. ( a ) We use an SLM to modulate the generated mode (left side) with the opposite-handed phase hologram (phase modulation shown in grey scale, linearly from 0=black to 2 π =white). The resulting intensities (right side) resemble the expected fundamental Gauss mode with an on-axis intensity maximum. However, a reduction of the modulated Gauss mode quality can be seen for higher orders. ( b ) We quantify these results by additional modulation of each generated mode (from −3rd order, dark blue, to 3rd order, dark green) with phase holograms of all neighbouring modes and coupling to a single-mode fibre (filtering higher-order modes). Thereby, we are able to measure the purity of the generated modes. We find that the expected OAM modes of a specific order are generated depending on the particular slit positions with high efficiency (highest bar for each slit position). The overlap with direct neighbouring modes is around 20%, which decreases down to <1% for third neighbours. The varying relative power for different orders stems from the Gaussian mode shape of the laser, through which the slit was moved. Full size image Interfacing high-dimensional path and OAM entanglement After characterization of the reversed MS as an interface between the lateral position and OAM, we demonstrate its use in quantum optical experiments and transform a bipartite path-entangled state to an OAM-entangled state, even for higher-dimensional states. We create pairs of orthogonally polarized, path-entangled photons from position correlation in a spontaneous parametric down-conversion process [2] , [28] , [29] ( Fig. 4a and Methods). 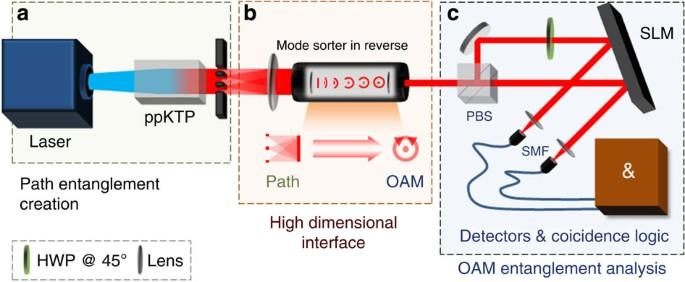Figure 4: Schematic of the experimental set-up to interface the high-dimensional path and OAM entanglement. (a) By pumping a non-linear crystal (ppKTP) with a 405-nm laser (blue) we create pairs of orthogonally polarized photons with 810 nm wavelength in a down-conversion process (red). A triple slit is placed directly behind the crystal. Both photons of a pair emerge together through one of the three slits. The final state is a superposition of the pair passing the three slits, hence the pair is entangled in the path. (b) A lens transforms the path entanglement to a transverse momentum entanglement, which is then transformed by the reversed mode sorter (black tube) to the OAM degree of freedom. (c) The OAM-entangled pair of photons is split by a polarizing beam splitter (PBS) and the vertically polarized photon is rotated by a half-wave plate (HWP) to the required polarization for phase modulation with the SLM. Each photon is filtered individually depending on its spatial mode, by a hologram displayed on a spatial light modulator (SLM) and by coupling to single-mode fibres (SMF). Avalanche photo-diode, single-photon detectors and a coincidence logic (brown box) are utilized to detect photon pairs and the observed correlations are subsequently analysed. By placing a triple slit directly behind (less than 1 mm) the crystal we filter out only three positions, which leads to an expected two-photon qutrit path-entangled state Figure 4: Schematic of the experimental set-up to interface the high-dimensional path and OAM entanglement. ( a ) By pumping a non-linear crystal (ppKTP) with a 405-nm laser (blue) we create pairs of orthogonally polarized photons with 810 nm wavelength in a down-conversion process (red). A triple slit is placed directly behind the crystal. Both photons of a pair emerge together through one of the three slits. The final state is a superposition of the pair passing the three slits, hence the pair is entangled in the path. ( b ) A lens transforms the path entanglement to a transverse momentum entanglement, which is then transformed by the reversed mode sorter (black tube) to the OAM degree of freedom. ( c ) The OAM-entangled pair of photons is split by a polarizing beam splitter (PBS) and the vertically polarized photon is rotated by a half-wave plate (HWP) to the required polarization for phase modulation with the SLM. Each photon is filtered individually depending on its spatial mode, by a hologram displayed on a spatial light modulator (SLM) and by coupling to single-mode fibres (SMF). Avalanche photo-diode, single-photon detectors and a coincidence logic (brown box) are utilized to detect photon pairs and the observed correlations are subsequently analysed. Full size image where S 1/2/3 denote the slit that both photons pass through and the subscripts H/V label their polarization. The amplitudes a , b and c ( a 2 + b 2 + c 2 =1) as well as the phases ϕ 1 and ϕ 2 are described by real numbers and depend on the pump beam behind each slit. Therefore, they are flexibly adjustable by modulating the intensity and phase of the pump beam. If only two slits are used a state is created that consists of the first two terms. The slits are placed in the focal plane of a lens followed by the reversed MS, which leads to a transformation of the path entanglement to the OAM degree of freedom. Thus, the total transformation acts as an interface between the high-dimensional path and spatial mode entanglement ( Fig. 4b ). In our experiment the distance between the three (two) slits corresponds to the 0th, −3rd and +3rd order LG modes (0th and −3rd order). We chose these three orders to reduce the earlier-demonstrated modal overlap of the MS to <1%. Hence the expected state can be written as where −3, 0 and 3 label the order of the mode or OAM quanta. The flexibility in adjusting the amplitudes, phases, OAM values and dimensionality of the state (via transmittance, positions and number of slits) implies a general method to custom-tailor high-dimensional OAM entanglement. To verify the OAM entanglement we split the transferred photon pair with a polarizing beam splitter and analyse each photon with a spatial mode filter. Again, we realize the filter by a combination of a phase hologram on the SLM and a single-mode fibre [10] , [26] . Single-photon detectors (avalanche diodes) together with a coincidence logic are used to register correlations between the two spatial modes of a pair ( Fig. 4c ). Measuring high-dimensional OAM entanglement We quantitatively demonstrate entanglement by using a simple, powerful entanglement witness that compares the extracted fidelity (overlap between an ideal state of equation (2) and the measured data) and the maximally expected fidelity for d -dimensional entangled states. If the measured fidelity exceeds the known bound for a d -dimensional entangled state, our results prove at least ( d +1)-dimensional entanglement (see Methods). In a first experiment, we test for qubit entanglement by measuring correlations between the 0th order (Gauss mode) and the −3rd order LG mode ( Fig. 5 ). From the measured maxima and minima of these correlation fringes, the visibilities can be deduced. The highest fidelity calculated from the visibilities in all mutually unbiased bases was 97±2% with an ideal state where a =0.54 and b =0.84. The maximum fidelity that would be achievable for separable states is 71%. 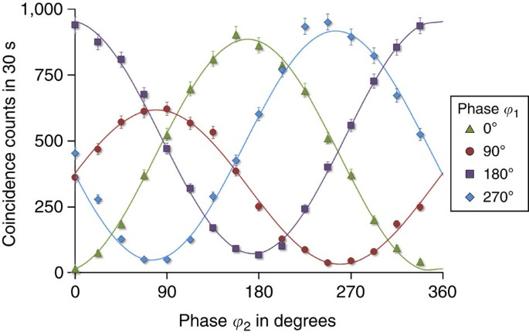Figure 5: Coincidence measurements to confirm the two-dimensional OAM entanglement. With the hologram displayed on the SLM we measured for each observed photon the superposition |−3›+eiϕ|0›, whereϕis an adjustable phase between 0° and 360°. We measured coincidence fringes for four different settings of the phaseϕ1of one photon, while the phaseϕ2setting for the partner photon is scanned in steps of 22.5°. The lines show the best sin2-fits that lead to visibilities of ~90%, confirming entanglement. For one setting (90°) the maximum is found to be significantly smaller than for the other phase settings. This might originate from a slight misalignment of the mode sorter. Error bars (if big enough to be seen) depict one sigma confidence with Poissionian count statistics assumed. Figure 5: Coincidence measurements to confirm the two-dimensional OAM entanglement. With the hologram displayed on the SLM we measured for each observed photon the superposition |−3›+ e iϕ |0›, where ϕ is an adjustable phase between 0° and 360°. We measured coincidence fringes for four different settings of the phase ϕ 1 of one photon, while the phase ϕ 2 setting for the partner photon is scanned in steps of 22.5°. The lines show the best sin 2 -fits that lead to visibilities of ~90%, confirming entanglement. For one setting (90°) the maximum is found to be significantly smaller than for the other phase settings. This might originate from a slight misalignment of the mode sorter. Error bars (if big enough to be seen) depict one sigma confidence with Poissionian count statistics assumed. Full size image In addition to the results of the entanglement witness, we used the measurements shown in Fig. 5 to test for two-dimensional entanglement with the popular criterion of a CHSH-Bell inequality [30] . For local realistic theories the following bound holds: where α , α ′, β and β ′ denote different measurement settings (phases of the measured superpositions) and E stands for the normalized expectation value for photon pairs to be found with this combination of modes. In our measurement we achieve a value of 2.47±0.04, which violates the classical bound by more than 10 standard deviations (Poissionian count statistics assumed). Both results confirm our observation of two-dimensional entanglement. In a second experiment we take advantage of all three implemented slits and test for OAM qutrit entanglement. Similar to earlier results [12] , [22] , the entanglement witness enables us to draw conclusions about the global dimensionality of the entanglement while restricting ourselves to qubit-subspace measurements. In our experiment this approach corresponds to the measurements of all visibilities in all two-dimensional subspaces that is for l -values of 0/−3, 0/+3 and −3/+3. The best statistical significance for genuine qutrit entanglement was found for an ideal state where a = c =0.48, b =0.73. Here, the fidelity obtained from the measured visibilities is 89±4%, which exceeds the upper bound for any two-dimensional entangled state (77%) by more than three standard deviations. Note that in both cases (qubit and qutrit entanglement) no background subtraction has been applied. Also, the largest amplitude was found for the Gauss mode because it corresponds to the central slit where the pump intensity and thus the down-conversion rate is maximal. Our set-up is not limited to qutrits but can be naturally extended to d -dimensional entanglement. A broader pump beam and a wider crystal in combination with a d -slits arrangement would lead to d possible paths and thus d -dimensional entanglement. A further way to increase the dimensionality of the path entanglement as well as the efficiency would be an arrangement with many integrated down-conversion crystals [31] in waveguide structures or fibre-coupled down-conversion crystals pumped in parallel [3] . In that case the waveguides or a fibre groove array could replace the multiple slits. Furthermore, it has been shown recently that the MS works for up to 50 states [32] and that the MS can be improved to reduce the overlap between neighbouring modes [27] . These improvements in MS design suggest that our approach can be readily extended to higher qudit entanglement. Although outside of the scope of the present work, it will be interesting to further investigate the detected higher-order radial structures, their potential as an additional dimension to encode information and their relation to the slit height. In addition, a suppression of the additional rings, by adapting the shape of the slit and improving the MS performance, might be crucial for the efficient interconnection of waveguide structures over long distances. In conclusion, we have shown that the MS in combination with a slit can be used, in reverse, to generate LG modes and their superpositions up to at least l =±10. Using fast switching techniques for optical paths the method can increase the switching rate between different LG beams in classical information technologies or LG-mode-based quantum cryptography applications. In addition, our results demonstrate a flexible way to create high-dimensional OAM entanglement. Most importantly, they show a way to implement an quantum interface between two approaches to high-dimensional quantum information: path encoding in waveguide structures for scalable, complex photonic quantum circuits including arbitrary unitary operation for higher-dimensional states [1] , [3] , and OAM encoding to distribute those high-dimensional quantum states [5] , [6] , [7] , [8] , [9] in a broad quantum network scenario. Creation of path-entangled photons To create correlated photons we used a cw 405-nm laser diode to pump a periodically poled potassium titanyl phosphate crystal (1 × 2 × 5 mm 3 ) with ~30 mW pump power. The pump beam diameter was ~1 mm (FWHM), which leads to a broad region where the two orthogonally polarized photons (Type II down-conversion) with 810 nm wavelength can be created. In the near-field of the crystal—directly behind it—the photons are correlated in the transverse spatial position [28] , [29] , that is, if one photon is found to be at a specific transverse spatial location the partner photon will be found ideally at exactly the same location too. This stems from the down-conversion process itself, where the pump photon generates two down-converted photons at some transverse spatial position of the crystal. Because the actual location of the down-conversion process is not determined, that is, it can happen everywhere within the pump beam spread, the generated photon pairs are in a superposition of all possible positions. A double or triple slit placed behind the crystal selects only two or three lateral positions; thus the photon pairs that pass the slits are in a superposition of two or three locations. In other words, they are in path-entangled qubit or qutrit states. For the multi-slit arrangement, the slits had a width of 150 μm and were separated by 250 μm, which resemble the dimensions typically used for telecom-standard fibre arrays. A schematic of the set-up can be seen in Fig. 4a . The presented scheme is readily extendable to more than three-dimensional entanglement, by increasing the number of slits. Furthermore, our source could be directly connected to complex integrated waveguide structures. Bipartite witness for d -dimensional entanglement We develop a witness framework requiring only measurements in two-dimensional subspaces. From these subspace measurements we compute the fidelity F of the experimentally produced state with a specially chosen high-dimensional state. We then use the techniques developed below to bound the maximal overlap of states with a bounded Schmidt rank d and the chosen high-dimensional state. If the subspace measurements reveal a higher overlap than this bound, the production of at least d +1-dimensional entanglement is proven. Construction of the witness proceeds as follows. The Schmidt decomposition of the assumed high-dimensional state can be written as , where i labels the different states (in our experiment the spatial modes), D denotes the dimension of the Hilbert space and the coefficients are chosen in a decreasing order, that is, λ 1 ≥ λ 2 ≥(...)≥ λ d (in the main text λ i corresponds to the amplitudes a , b and c ). This choice has the advantage that , where all appearing matrix elements can be determined by three visibility measurements in two-dimensional subspaces, the number of which scales as the square root of those required for a full-state tomography. We can now construct a witness for d -dimensional entanglement (Schmidt number witness) by comparing the two fidelities and where ρ labels the density matrix related to our measurements and | ϕ d › denotes states with a bounded Schmidt rank d . If equation F > f d holds, the measurements cannot be explained by a d -dimensional entangled state; thus, the generated bipartite system was (at least) genuinely ( d +1)-dimensionally entangled. Calculation of the maximal fidelity for d -entangled states proceeds in the following manner. The maximization in equation (5) runs over all states with at most d -dimensional entanglement (Schmidt rank d ). This maximal overlap between and the guessed state | ψ › (expressed in terms of the Schmidt coefficients) can be rewritten as By rearranging the terms and introducing the operator B = c kl | k ›‹ l | and the rank d -projector P d B *= B * (which always exists if B * is of rank d , as | ϕ d › is of Schmidt rank d ), we get and since the trace is invariant under cyclic permutations we can write Using the Cauchy–Schwarz inequality for the Hilbert–Schmidt inner product (for the inner product ‹ A , B ›:=Tr( AB † ) it reads |‹ A , B ›| 2 ≤‹ A , A ›‹ B , B ›), we get the inequality Because and choosing the obviously maximizing we get the upper bound for the fidelity of d -dimensional entangled states of By choosing we find that , thus proving that our bound is indeed tight, that is, The inequality for the witness of d -dimensional entanglement follows from the above. Hence, from the visibility measurements in all two-dimensional subspaces we can now reveal information about the global dimensionality of the bipartite entanglement. If the following inequality holds, we have proven that our measurement results can only be explained by an at least ( d +1)-dimensionally entangled state: Note that although we have derived the proof by assuming a pure state the witness holds even for mixed states because they would only lower the bound (due to the convexity of the fidelity). Thus, the presented witness is a state-independent test for high-dimensional entanglement. How to cite this article: Fickler, R. et al. Interface between path and orbital angular momentum entanglement for high-dimensional photonic quantum information. Nat. Commun. 5:4502 doi: 10.1038/ncomms5502 (2014).